Re-evaluating the evidence for a universal genetic boundary among microbial species 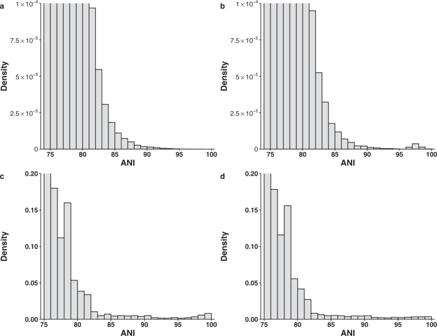Fig. 1: Distribution of ANI values. Top panel: from the phylogenetic simulations.aComparisons between 3000 taxa simulated using a phylogenetic tree with 3000 tips and a constant rate of diversification.bComparisons in the same dataset except that 30 of 3000 taxa each have two very closely related genomes sequenced. Bottom panel: from genomes subsampled from the 90K genome dataset.cTwo genomes were randomly selected from each of the 397 named species with ≥10 genomes.dTwo phylogenetic representative genomes were selected for each of the 397 named species with ≥10 genomes. 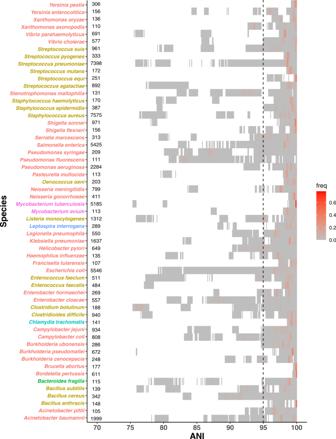Fig. 2: The distribution of ANI for 61 named species with ≥100 genomes in the 90K genome dataset. Each block represents a bin of ANI values between pairs of genomes within the same species and is colored by the ANI density in the bin. Species are colored by phylum. The numbers next to the species names are the numbers of genomes in the 90K dataset for the species. The vertical dotted line represents the 95% ANI threshold. Genome datasets Two genome datasets were used in this study. The first is the 90K genome dataset from the original paper [1] . It contains both complete and draft bacterial and archaeal genomes. The second dataset consists of 10,616 complete bacterial genomes downloaded from the NCBI RefSeq database on September 6, 2018 (10K genome dataset). From each genome in the 10K dataset, we identified 31 universal protein-coding marker genes using AMPHORA2 [15] and constructed a bacterial genome tree based on the concatenated and trimmed protein sequence alignment of the marker genes using FastTree [16] . Treemmer (version 0.3) [17] was used to choose 3000 representative genomes that maximized the phylogenetic diversity in the 10K genome dataset. Average nucleotide identity (ANI) The ANI values for the 90K genome dataset were downloaded from the original study. For the 10K genome dataset, the 3000 representative genomes were compared against the full 10K dataset using FastANI (version 1.2). Modeling the relationship between branch length and ANI The 3000 representative genomes were used to model the empirical relationship between ANI and branch length. The median of ANI was calculated across binned branch lengths (bin width: 0.05 substitution/site) to use as the actual data to fit the relationship between ANI and branch length l through the function \(ANI( \% )=k+\frac{\alpha \cdot (100-k)}{{l}^{s}+\alpha }\) , where k , s and α are shape parameters to be estimated. Minimization of the sum of squares error was performed using the optim function in R. The best fit parameters for our data are α = 0.075, k = 73.94, and s = 0.63. Branch lengths >2.5 substitutions/site were removed because of the lack of data points. Simulation of continuous genetic diversity and biased within-species sampling The rtree function in the ape package in R was used to simulate a random phylogenetic tree of 3000 tips, with its branch lengths following an exponential distribution with a constant rate of 19.2, estimated from the genome tree of the 3000 representative genomes. Using the formula described above, the ANI value between a pair of genomes was computed from the branch length between them. To simulate biased sampling within species, a random tip was chosen and two descendants were added to that tip, with the branch length from the tip to the descendant sampled from the same exponential distribution, but its value restricted to the bottom 1% of the distribution. This procedure was repeated on the remaining 2999 tips until n tips were processed. Each simulation was run with ten replicates. Assessing the within-species sampling bias Species with ≥10 genomes were selected from the 10K genome dataset. For each species, a subtree compiling the respective genomes was extracted from the full phylogeny of 10,616 genomes and Treemmer was used to iteratively remove one tip of the tip-pair with the shortest branch length until three tips remained. The remaining total branch length of the tree was divided by the total branch length of the initial tree to calculate the relative tree length at each iteration. Rickettsia japonica and Chlamydia muridarum were removed from this analyses because their genomes have identical marker sequences and branch lengths equal to zero. To further evaluate the within-species sampling bias, we tested how much known genetic diversity is recovered by the complete genomes, using E. coli as an example. We extracted 868 unique 16S rRNA gene sequences with no ambiguous bases from 602 complete E. coli genomes in the 10K genome dataset and BLAST searched them against 8655 E. coli 16S rRNA gene sequences from the GreenGene 13.8 database. A match was defined as a pair of sequences with 100% identity for their entire sequences. The matched GreenGene 16S rRNA sequences were then mapped to the 99% OTUs (operational taxonomic units) of the GreenGene database. The total branch length covered by the mapped OTUs in the 16S rRNA tree of 44 E. coli 99% OTUs was calculated to estimate the coverage of E. coli diversity by complete genomes. Subsampling of two genomes For named species with ≥10 genomes in the 90K dataset, two genomes were sampled from each species either randomly or by selecting the pair with the lowest ANI value. Among all pairwise comparisons within the species, the pair with the lowest ANI best represents the phylogenetic diversity of the species. Benchmark the performance using 95% ANI for species demarcation Using the 3000 representative genomes as the query, we ran FastANI against the full 10K genome dataset. For each query genome, the subject genome with the maximum ANI value was used to benchmark the performance of using the 95% ANI threshold to demarcate bacterial species. A true positive is a query-subject pair belonging to the same species and having an ANI ≥ 95%. A false positive is a genome pair of different species with an ANI ≥ 95%, and a false negative is a genome pair of the same species with an ANI < 95%. Precision was calculated by: the number of true positive/(number of true positive + number of false positive) and recall was calculated by: the number of true positive/(number of true positive + number of false negative). Reporting summary Further information on research design is available in the Nature Research Reporting Summary linked to this article.